Tumour microvesicles contain retrotransposon elements and amplified oncogene sequences Tumour cells release an abundance of microvesicles containing a selected set of proteins and RNAs. Here, we show that tumour microvesicles also carry DNA, which reflects the genetic status of the tumour, including amplification of the oncogene c-Myc . We also find amplified c-Myc in serum microvesicles from tumour-bearing mice. Further, we find remarkably high levels of retrotransposon RNA transcripts, especially for some human endogenous retroviruses, such as LINE-1 and Alu retrotransposon elements, in tumour microvesicles and these transposable elements could be transferred to normal cells. These findings expand the nucleic acid content of tumour microvesicles to include: elevated levels of specific coding and non-coding RNA and DNA, mutated and amplified oncogene sequences and transposable elements. Thus, tumour microvesicles contain a repertoire of genetic information available for horizontal gene transfer and potential use as blood biomarkers for cancer. Increasing knowledge of the genetic and epigenetic changes occurring in cancer cells provides an opportunity to detect, characterize and monitor tumours by analysing tumour-related nucleic acid sequences and profiles. Cancer-related changes include specific mutations in gene sequences [1] , [2] , up- and downregulation of messenger RNA (mRNA) and microRNA (miRNA) expression [3] , [4] , mRNA splicing variations and changes in DNA methylation patterns [5] , [6] , as well as amplification and deletion of genomic regions [7] . Brain tumours comprise a variety of phenotypic and genetic subtypes and knowing the expression/mutational profile of individual cancers is critical for personalized medicine as many drugs target specific pathways affected by the genetic status of the tumours. Detection of genetic biomarkers in tumour patient blood samples is challenging because of the need for high sensitivity against a background of normal cellular DNA/RNA found circulating in blood. Microvesicles released by tumour cells into the circulation can provide a window into the genetic status of individual tumours [8] , [9] . Many types of cancer cells release an abundance of small membrane-bound vesicles, which have been observed on their surface in culture [8] , [10] . These microvesicles are generated and released through several processes and vary in size (30 nm to 1 μm in diameter) and content [11] . Microvesicles can bud/bleb off the plasma membrane of cells, much like retrovirus particles [12] , be released by fusion of endosomal-derived multivesicular bodies with the plasma membrane [13] , or be formed as apoptotic bodies during programmed cell death [14] . In addition, defective retrovirus particles derived from human endogenous retroviral (HERV) elements may be found within microvesicle populations [15] . Different microvesicle types often co-purify and given the evolving nomenclature for these various types, our study has focused on collective microvesicle populations of <0.22 μm in diameter. Microvesicles from various cell sources have been extensively studied with respect to protein and lipid content [16] , [17] . They also contain a select set of cellular RNAs and mitochondrial DNA [8] , [18] , [19] , [20] and may facilitate the transfer of genetic information between cells and/or act as a 'release hatch' for DNA/RNA/proteins that the cell is trying to eliminate. Both mRNA and miRNA in microvesicles can be functional following uptake by recipient cells [8] , [19] , [21] , [22] , [23] , [24] and it has also been shown that apoptotic bodies can mediate horizontal gene transfer between cells [25] . Increased transcription of retrotransposon elements in the human genome has been noted in a number of cancer cell types. These repetitive elements constitute almost 50% of the human genome and include: half a million LINE-1 (L1) elements, of which about 100 are transcriptionally active and encode proteins involved in retrotransposition, including reverse transcriptase (RT) and integrase; a million Alu elements, which depend on L1 functions for integration; and thousands of provirus HERV sequences, some of which contain near-to-full-length coding sequences [15] , [26] . Increased expression of retrotransposon elements in cancer seems to result in part from overall hypomethylation of the genome, which is also associated with genomic instability [27] , [28] and tumour progression [29] , [30] . Interestingly, increased expression of L1 and HERV RNA and proteins, as well as formation of retrovirus-like particles, have been reported in tumour tissue from breast cancer, melanoma and germ cell carcinoma [31] , [32] , [33] . Retrotransposon RNA/proteins, as well as antibodies against HERV proteins and virus-like particles, are also found in blood of some cancer patients [33] , [34] , [35] , [36] . In this study, we examined the nucleic acid content of microvesicles released by cells in culture and tumours in vivo in: glioblastoma (GBM), the most common and malignant brain tumour in adults; medulloblastoma, the most common and malignant tumour in children with frequent amplification of c-Myc [37] and atypical teratoid rhabdoid tumour (AT/RT), a high-grade malignant tumour in children [38] . We also included a peripheral tumour: malignant melanoma, one of the most common cancers, which can metastasize to the brain [39] . Epidermoid carcinoma tumour cells were used as a control for the in vivo study, as they have amplified epidermal growth factor receptor (EGFR), but not c-Myc genes [40] . We examined the nucleic acid content of microvesicles released by cells in culture and tumours in vivo . In addition to RNA, tumour microvesicles contain single-stranded DNA (ssDNA; exoDNA, ex creted o ut of cells in microvesicles), including both genomic and cDNA, as well as high levels of transposable elements. Medulloblastoma cells with the amplified oncogene c-Myc had higher DNA/RNA levels of this oncogene in the microvesicles compared with cells without c-Myc amplification. Elevated human c-Myc RNA was also found in microvesicles isolated from mice-bearing tumours with amplified c-Myc. Further, an abundance of retrotransposon RNA, including HERV, L1 and Alu sequences was found in tumour-derived microvesicles. Tumour microvesicles contain amplified genomic DNA (gDNA), cDNA and retrotransposon elements that may have a role in genetic communication between cells and provide a potential source of tumour biomarkers. Cultured cells release an abundance of microvesicles We characterized the size distribution and amount of microvesicles released from tumour cells and normal fibroblasts in culture using Nanosight LM10 nanoparticle tracking analysis ( Fig. 1 ). Medulloblastoma cells were found to release more microvesicles per cell than the other cells types analysed (13,400–25,300 per cell per 48 h for medulloblastomas and 7,000–13,000 per cell per 48 h for the GBM and melanoma cells). Normal human fibroblasts released 3,800–6,200 per cell per 48 h, were of low passage and grew with similar rates as the tumour lines in culture, but of larger size and hence greater surface area per cell. Levels of RNA in microvesicles (exoRNA) from tumour cells as compared with normal fibroblasts were 120- to 310-fold higher for medulloblastoma cells and 2.8- to 6.5-fold higher for GBM cells, with melanoma cells having similar levels of exoRNA compared with fibroblasts despite shedding more than twice as many microvesicles. Thus, medulloblastoma tumour cells, in particular, release abundant microvesicles with a high content of exoRNA. 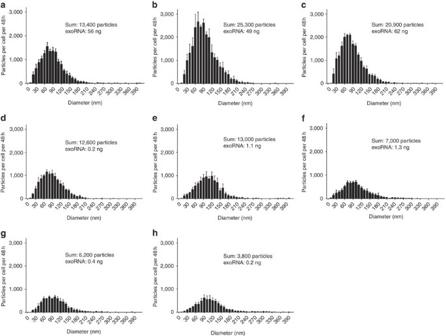Figure 1: Analysis of microvesicle profiles and RNA yields from different human cell lines. Microvesicles were isolated from three medulloblastoma cell lines (a, D384,b, D425 andc, D458), one melanoma (d, Yumel 0106), two GBMs (e, 20/3 andf, 11/5) and two normal fibroblasts (g, HF19 andh, HF27) and measured with Nanoparticle Tracking Analysis (NanoSight). The number of particles per cell per 48 h is shown on theyaxis, and the size distribution (particle diameter) on thexaxis. The sum refers to the total number of particles released per cell over 48 h and the exoRNA refers to the total microvesicle RNA yield per 1×106cells per 48 h. The results are presented as the mean±s.e.m. (n=3). Figure 1: Analysis of microvesicle profiles and RNA yields from different human cell lines. Microvesicles were isolated from three medulloblastoma cell lines ( a , D384, b , D425 and c , D458), one melanoma ( d , Yumel 0106), two GBMs ( e , 20/3 and f , 11/5) and two normal fibroblasts ( g , HF19 and h , HF27) and measured with Nanoparticle Tracking Analysis (NanoSight). The number of particles per cell per 48 h is shown on the y axis, and the size distribution (particle diameter) on the x axis. The sum refers to the total number of particles released per cell over 48 h and the exoRNA refers to the total microvesicle RNA yield per 1×10 6 cells per 48 h. The results are presented as the mean±s.e.m. ( n =3). Full size image Characterization of RNA and DNA in microvesicles Isolated microvesicles were treated extensively with DNase before nucleic acid extraction to reduce the chance of external DNA contamination (external RNase treatment did not affect the RNA yield, indicating no external RNA). After microvesicle lysis and nucleic acid purification, the exoRNA fraction was DNase treated and the exoDNA fraction was RNase treated. The RNA profile varied among cell types and culture conditions, but in general, RNA with intact 18S and 28S ribosomal peaks was isolated from microvesicles ( Supplementary Fig. S1 ). ExoDNA was more abundant in microvesicles from tumour as compared with normal cells, and appeared to be primarily single stranded. When exoDNA from medulloblastoma tumour cells (D384) was analysed using a double-stranded DNA detection chip, no DNA was detected ( Supplementary Fig. S2a ). However, when this exoDNA was subjected to second strand synthesis, this same chip detected abundant double-stranded DNA ( Supplementary Fig. S2b ). The same experiment was performed on GBM cells (GBM 20/3) with similar results. The predominance of ssDNA in exoDNA was also confirmed by its complete sensitivity to S1 exonuclease digestion ( Supplementary Fig. S3 ). c-Myc oncogene amplification is reflected in exoRNA and exoDNA The levels of c-Myc amplification were measured at the genomic level (gDNA) by quantitative PCR (qPCR; Fig. 2a ). All three medulloblastoma cell lines had a significant amplification of c-Myc sequences (16- to 34-fold) compared with normal fibroblasts and other tumour cell types. RNA and DNA were extracted from microvesicles shed by these cell lines and measured by quantitative reverse transcription PCR (qRT-PCR) and qPCR, respectively, using primers in exon 3 ( Supplementary Table S1 ). The values for c-Myc sequences were normalized to glyceraldehyde 3-phosphate dehydrogenase ( GAPDH ), a housekeeping gene constitutively expressed in cells and found in exoRNA [8] and here in exoDNA. Microvesicles from all medulloblastoma cell lines showed elevated levels of c-Myc sequences, both for exoRNA (8- to 45-fold) and exoDNA (10- to 25-fold), compared with microvesicles from fibroblasts and tumour cells with diploid c-Myc copy numbers ( Fig. 2b,c ). Also, using primers that span a full intron, we successfully detected a 1.6 kbp fragment corresponding to the unspliced c-Myc gDNA (verified by sequencing) in exoDNA from all three medulloblastoma cell lines, but not in any of the other cell lines. Furthermore, to establish that this genomic fragment of c-Myc in microvesicles was derived from a genomic amplicon, we verified the presence of elevated levels of a flanking gene, POU5F1B gene [41] (PCR product also verified by sequencing) at levels matching those of c-Myc ( Supplementary Fig. S4 ). Levels of n-Myc sequences in cellular gDNA or exoRNA were also measured by qPCR and qRT-PCR and none of the tumour types showed genomic amplification of n-Myc sequences or elevated levels of n-Myc exoRNA ( Supplementary Fig. S5a,b ). 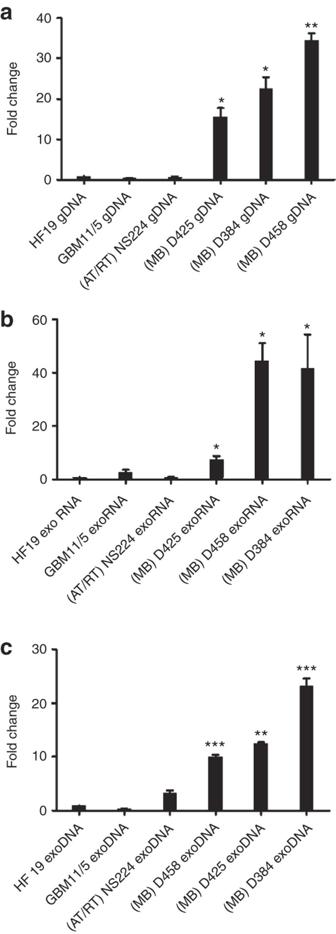Figure 2: Medulloblastomas with amplifiedc-Myconcogenes have elevatedc-MycexoRNA and exoDNA in their microvesicles. (a)c-Mycamplification levels were quantified in genomic DNA (gDNA) from one normal human fibroblast line (HF19), one GBM line (11/5), one atypical teratoid rhabdoid tumour (AT/RT) line (NS224) and three medulloblastoma (MB) lines (D425, D458 and D384). ExoRNA and exoDNA were also isolated from their corresponding microvesicles. (b) qRT-PCR and (c) qPCR were carried out on nucleic acid from microvesicles from the same cell lines to measure exoRNA and exoDNA, respectively.c-Myclevels were normalized toGAPDHin the same preparation and expressed as fold increase relative to normal fibroblasts. In all cases, values are expressed as mean±s.e.m. (n=3) and analysed by two-tailedt-test comparing MB lines to HF19 (*P< 0.05, **P<0.01, ***P<0.001). Figure 2: Medulloblastomas with amplified c-Myc oncogenes have elevated c-Myc exoRNA and exoDNA in their microvesicles. ( a ) c-Myc amplification levels were quantified in genomic DNA (gDNA) from one normal human fibroblast line (HF19), one GBM line (11/5), one atypical teratoid rhabdoid tumour (AT/RT) line (NS224) and three medulloblastoma (MB) lines (D425, D458 and D384). ExoRNA and exoDNA were also isolated from their corresponding microvesicles. ( b ) qRT-PCR and ( c ) qPCR were carried out on nucleic acid from microvesicles from the same cell lines to measure exoRNA and exoDNA, respectively. c-Myc levels were normalized to GAPDH in the same preparation and expressed as fold increase relative to normal fibroblasts. In all cases, values are expressed as mean±s.e.m. ( n =3) and analysed by two-tailed t -test comparing MB lines to HF19 (* P < 0.05, ** P <0.01, *** P <0.001). Full size image The levels of c-Myc DNA quantified for gDNA and exoDNA/RNA in these medulloblastoma lines were also compared with levels estimated by 250K single-nucleotide polymorphism (SNP) analysis ( Table 1 ; see Supplementary Fig. S5c for a representative heat map). The copy number of c-Myc was increased in medulloblastoma lines and was normal in the AT/RT tumour line. The increased levels of c-Myc exoDNA and exoRNA corresponded well to the genomic copy number estimated by 250k SNP and qPCR in the medulloblastoma cell lines. The normal diploid cell lines showed no amplification of c-Myc on exoRNA or exoDNA. To assess the potential diagnostic utility of using exoRNA to detect c-Myc amplification in tumours, human medulloblastoma cells ( c-Myc amplified) and epidermoid carcinoma tumour cells (non-amplified; Fig. 3a ) were grown as xenograft tumours in nude mice. Microvesicles were isolated from serum samples in tumour-bearing mice and human c-Myc exoRNA was detected in 2/5 (40%) of the medulloblastoma-bearing mice and in 0/5 of the epidermoid carcinoma-bearing mice ( Fig. 3b ). Table 1 Assessment of c-Myc gene amplification levels in different cell types. 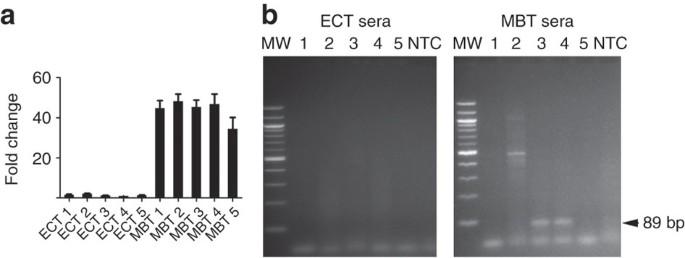Figure 3: Detection of amplified c-Myc sequences in serum microvesicles from tumour-bearing mice. Medulloblastoma (MBT; D425) and epidermoid carcinoma (ECT; A431) cells were used to generate subcutaneous tumours with and without c-Myc amplification, respectively. (a)c-Mycamplification was evaluated on all tumour samples at the RNA level after tumour resection. Values were normalized toGAPDH, presented as fold change compared with epidermoid carcinoma and shown as mean±s.e.m. (n=3). (b) ExoRNA was extracted from serum samples from five MBT and five ECT (MBT 1–5 and ECT 1–5, respectively).c-MycPCR product was amplified using human specific primers. Amplified DNA was resolved by electrophoresis in a 2% agarose gel and visualized with ethidium bromide staining.c-Mycis shown as an 89 bp fragment (arrow). MW, molecular weight; NTC, no template control. Full size table Figure 3: Detection of amplified c-Myc sequences in serum microvesicles from tumour-bearing mice. Medulloblastoma (MBT; D425) and epidermoid carcinoma (ECT; A431) cells were used to generate subcutaneous tumours with and without c-Myc amplification, respectively. ( a ) c-Myc amplification was evaluated on all tumour samples at the RNA level after tumour resection. Values were normalized to GAPDH , presented as fold change compared with epidermoid carcinoma and shown as mean±s.e.m. ( n =3). ( b ) ExoRNA was extracted from serum samples from five MBT and five ECT (MBT 1–5 and ECT 1–5, respectively). c-Myc PCR product was amplified using human specific primers. Amplified DNA was resolved by electrophoresis in a 2% agarose gel and visualized with ethidium bromide staining. c-Myc is shown as an 89 bp fragment (arrow). MW, molecular weight; NTC, no template control. Full size image Tumour microvesicles are enriched for retrotransposon elements Microarray analysis of cellular RNA and exoRNA sequences from a low-passage GBM line indicated high transcription levels of several retrotransposon sequences as evaluated using a whole-genome array. This data is represented on MA plots [42] as the cumulative abundance (in cells and microvesicles) of specific RNAs ( x axis) and the relative ratio of these RNAs in microvesicles versus cells ( y axis; Fig. 4a ). The axis scale is log 2 , so RNAs above 4 or below –4 on the y axis have at least 16-fold different levels in the microvesicles versus donor cells. Although RNA from DNA transposons was similar in content in cells and microvesicles ( Fig. 4b ), RNA from retrotransposons, for example, HERV, Alu and L1, was frequently higher in microvesicles than cells ( Fig. 4c–e ). This was particularly notable for the HERV sequences. HERV-H was the most abundant and microvesicle enriched in these GBM cells, followed by HERV-C, HERV-K6 and HERV-W ( Fig. 4f ). As only a selected subset of transposon/retrotransposon probes are represented on the Agilent arrays, this should be viewed as a partial screen. However, this array analysis supports selective packaging of retrotransposon RNA sequences, especially of HERV, in tumour microvesicles. 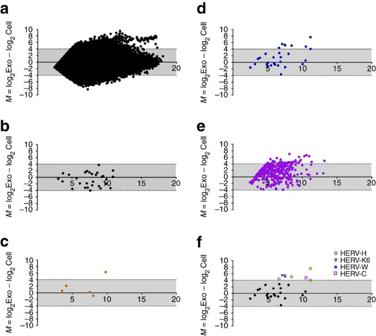Figure 4: GBM microvesicles are enriched for retrotransposon elements. The levels of transposon and retrotransposon sequences were compared with the rest of the RNA transcriptome in cells and microvesicles. ExoRNA and cellular RNA were isolated from GBM 20/3 cells and analysed on an Agilent two-color 44k array. (a) Relative levels of all represented RNA sequences (44,000 RNA probes) in cells and microvesicles were evaluated with an MA plot;yaxisM=log2Exo–log2Cell,xaxisA=0.5× (log2Exo+log2Cell). RNA intensities from capture probes aligning to (b) DNA transposons, (c) L1, (d) HERV and (e) Alu sequences were extracted and plotted on separate MA plots. (f) Identification of members of the HERV families enriched more than 16-fold in the microvesicles (M≥4). Some HERV families are represented more than once on the array. Figure 4: GBM microvesicles are enriched for retrotransposon elements. The levels of transposon and retrotransposon sequences were compared with the rest of the RNA transcriptome in cells and microvesicles. ExoRNA and cellular RNA were isolated from GBM 20/3 cells and analysed on an Agilent two-color 44k array. ( a ) Relative levels of all represented RNA sequences (44,000 RNA probes) in cells and microvesicles were evaluated with an MA plot; y axis M =log 2 Exo–log 2 Cell, x axis A =0.5× (log 2 Exo+log 2 Cell). RNA intensities from capture probes aligning to ( b ) DNA transposons, ( c ) L1, ( d ) HERV and ( e ) Alu sequences were extracted and plotted on separate MA plots. ( f ) Identification of members of the HERV families enriched more than 16-fold in the microvesicles (M≥4). Some HERV families are represented more than once on the array. Full size image As L1 and HERV-K retrotransposons, as well as Alu elements [26] , have been implicated in tumour progression, we further assayed their levels in cellular RNA and exoRNA from tumour and normal cells by qRT-PCR (again with the caveat that the primers do not detect all of the many variants of L1, ALU and HERV-K sequences), with levels normalized to GAPDH mRNA ( Fig. 5a–c ). L1 and Alu sequences were abundant in both cells and microvesicles and enriched in most of the microvesicles compared with the cells ( y >0; Fig. 5a,b ). The levels of retrotransposon sequences tended to be higher in exoRNA when compared with cellular RNA, with HERV-K being especially high in some tumours. Interestingly, HERV-K RNA was not detectable in exoRNA from normal human fibroblasts (HF19), so the microvesicle to cell ratio was calculated giving the exoRNA an arbitrary Ct value of 36 (below detection limit; Fig. 5c ). The enrichment ratio is not the same as abundance of the RNA. The three medulloblastoma cell lines had the highest abundance of HERV-K RNA in the microvesicles, but also in the cells (as shown by the high x axis value on the MA plot in Supplementary Fig. S6 ), making the enrichment ratio lower, especially for the D384 cells. To determine whether microvesicles could transfer HERV-K RNA to normal cells, human umbilical vein endothelial cells (HUVECs) were exposed to microvesicles from medulloblastoma cells and levels of HERV-K RNA were measured in the recipient HUVECs over time, showing efficient uptake with levels remaining high for at least 72 h after exposure ( Fig. 5d ). 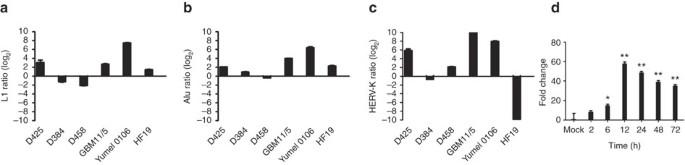Figure 5: Microvesicles are enriched in retrotransposon elements and can mediate horizontal gene transfer. Retrotransposon elements were quantified in cell RNA and exoRNA from three medulloblastoma (D425, D384 and D458), one GBM (11/5), one melanoma (0106) and one human fibroblast (HF19) line. The ratio of RNA abundances for (a) L1, (b) Alu and (c) HERV-K in microvesicles versus cells is shown, with RNA levels normalized to the housekeeping geneGAPDH. The relative ratios are presented as the average±s.e.m. (n=3–6). Enrichment of retrotransposons in either cells (y<0) or microvesicles (y>0) is expressed as log2values. (d) HUVECs were exposed to medulloblastoma microvesicles (D384) and their expression level of HERV-K RNA (normalized toGAPDH) was analysed by qRT-PCR over 72 h following exposure and plotted as fold change compared with non-infected cells (MOCK).P-values were calculated using the two-tailedt-test, comparing levels to MOCK infected cells (*P<0.05, **P<0.01). Figure 5: Microvesicles are enriched in retrotransposon elements and can mediate horizontal gene transfer. Retrotransposon elements were quantified in cell RNA and exoRNA from three medulloblastoma (D425, D384 and D458), one GBM (11/5), one melanoma (0106) and one human fibroblast (HF19) line. The ratio of RNA abundances for ( a ) L1, ( b ) Alu and ( c ) HERV-K in microvesicles versus cells is shown, with RNA levels normalized to the housekeeping gene GAPDH . The relative ratios are presented as the average±s.e.m. ( n =3–6). Enrichment of retrotransposons in either cells ( y <0) or microvesicles ( y >0) is expressed as log 2 values. ( d ) HUVECs were exposed to medulloblastoma microvesicles (D384) and their expression level of HERV-K RNA (normalized to GAPDH ) was analysed by qRT-PCR over 72 h following exposure and plotted as fold change compared with non-infected cells (MOCK). P- values were calculated using the two-tailed t -test, comparing levels to MOCK infected cells (* P <0.05, ** P <0.01). Full size image ExoDNA was also analysed at the retrotransposon level with qPCR. The levels of L1, ALU and HERV-K DNA were measured on nuclear gDNA isolated from the cells and compared with the exoDNA level in the corresponding microvesicles (with levels normalized to GAPDH ). The exoDNA (presumably originating from the cytoplasmic compartment) and gDNA (isolated from the nuclear compartment of the cells) showed clearly different abundance patterns ( y ≠0). L1 was slightly enriched in all medulloblastoma microvesicles, whereas Alu was not ( Fig. 6a,b ) and two of the medulloblastomas (D425 and D384) were enriched in HERV-K DNA ( Fig. 6c ). Interestingly, the enrichment of the transposable elements at the exoDNA level in the medulloblastoma cell lines corresponded to high levels of endogenous RT activity in exosomes ( Fig. 6d ), suggesting that a fraction of exoDNA may be cDNA. By comparison, Yumel 0106 and GBM11/5 cells had very little L1 and HERV-K exoDNA in the microvesicles compared with the cells (as shown by the negative values on the bar graph in Fig. 6a,c ). As the exoDNA yield in microvesicles was decreased by about 50% following inhibition of DNA replication with mimosine ( Supplementary Fig. S7 ), it seems that some of the exoDNA may also be fragments of gDNA generated during DNA replication and mitosis [45] . 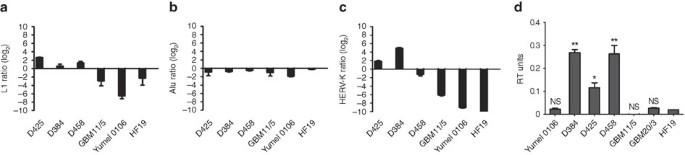Figure 6: Retrotransposon DNA sequences in microvesicles. Cellular and microvesicle DNA was isolated from three medulloblastoma (D425, D384 and D458), one GBM (11/5), one melanoma (0106) and one human fibroblast (HF19) line. qPCR analysis was carried out for (a) L1, (b) Alu and (c) HERV-K in gDNA and exoDNA. Ct values were normalized toGAPDHlevels and are shown as relative enrichment of transposons in cells (y<0) and microvesicles (y>0). (d) RT activity was measured in the microvesicles using the EnzChek RT Assay Kit (Invitrogen) and normalized to protein content. Results are expressed as average±s.e.m. (n=3). (*P<0.05, **P<0.01); NS=not significantly different from HF19). Figure 6: Retrotransposon DNA sequences in microvesicles. Cellular and microvesicle DNA was isolated from three medulloblastoma (D425, D384 and D458), one GBM (11/5), one melanoma (0106) and one human fibroblast (HF19) line. qPCR analysis was carried out for ( a ) L1, ( b ) Alu and ( c ) HERV-K in gDNA and exoDNA. Ct values were normalized to GAPDH levels and are shown as relative enrichment of transposons in cells ( y <0) and microvesicles ( y >0). ( d ) RT activity was measured in the microvesicles using the EnzChek RT Assay Kit (Invitrogen) and normalized to protein content. Results are expressed as average±s.e.m. ( n =3). (* P <0.05, ** P <0.01); NS=not significantly different from HF19). Full size image Previous studies have shown that microvesicles released from tumour cells into the blood stream of cancer patients contain a representation of the tumour transcriptome, including characteristically high levels of some mRNAs and miRNAs, and mutant/splice variant mRNAs, as well as tumour-related proteins [8] , [9] , [43] , [44] . We now find that microvesicles derived from cultured tumour cells also contain high levels of exoDNA—predominantly ssDNA fragments. Interestingly, exoDNA was virtually undetectable in normal skin fibroblasts used in this study. Of the tumour lines evaluated, both exoDNA and exoRNA were highest in microvesicles from medulloblastoma cells, which had genomic amplification and high-expression levels of the c-Myc oncogene. In addition, tumour microvesicles were found to be highly enriched in certain retrotransposon RNA sequences, especially for some of the HERVs. Interestingly, some of the tumour cell types also had enriched levels of exoDNA for transposable elements (primarily L1 and HERV). We also found that exosomes have RT activity, especially from the medulloblastomas, indicating that some of the exoDNA transposable elements may represent cDNAs. It has previously been shown that reverse transcribed transposable element cDNA is normally degraded by the Trex1 protein, a 3′-exonuclease that functions as an intrinsic cell protection mechanism. If Trex1 protein is knocked out, ssDNA accumulates in the cytoplasm, especially L1, HERV and Alu ssDNA [45] . Because microvesicles are sticky and can bind free-floating gDNA on their surface [46] , intact microvesicles were treated extensively with DNAse before analysis of exoDNA contained within them. Apoptotic vesicles, which are typically larger than the microvesicle fraction we analysed (<0.2 μm), could also potentially contribute gDNA into the exoDNA fraction. To evaluate this contribution we incubated cells with an apoptosis-inducing agent, doxorubicin. Surprisingly, this led to a reduction in exoDNA yield, indicating that cells undergoing apoptosis shed fewer microvesicles than healthy cells (data not shown). In addition, the bar graphs of transposable element DNA ( Fig. 6a–c ) showed differential levels in microvesicles versus the cells from which they were derived ( y ≠0), indicating a different composition of exoDNA compared with nuclear DNA. The elevated c-Myc exoDNA levels in microvesicles from medulloblastoma cells with amplified c-Myc could have several potential sources. They may arise from extra-genomic copies of the amplified c-Myc gene region, which are typically 0.1–1 Mbp and contain one or more origins of DNA replication [47] . These amplified sequences can appear cytogenetically as small 'double minute' chromosomes, which can end up in the cytoplasm during mitosis or be eliminated by extrusion out of cells within micronuclei [48] . Fragments of these double minute chromosomes may end up in microvesicles as supported by the presence of c-Myc intronic and flanking gene sequences. In addition, ssDNA in the cytoplasm and microvesicles may arise during abnormal replication of DNA in cancer cells through faulty re-replication and accumulation of short Okazaki fragments of linear ssDNA [49] . This potential source is supported by results from treatment with mimosine, which blocks DNA replication in late G1 and reduced exoDNA levels in a dose-dependent manner. Further, some of the exoDNA may be derived from reverse transcription of cellular RNAs, as supported by the RT activity in microvesicles. Retrotransposable elements can create a dynamic aspect to the genome, with new insertions of retrotransposon and cDNA sequences potentially leading to mutations, deletions, rearrangements and changes in gene expression. Genome stability is maintained in normal differentiated cells by suppressed transcription of these retrotransposon elements, with tumour cells frequently having elevated retrotransposon expression [27] . The specific HERV type found in tumour microvesicles may depend on the cell of origin of the tumour. The abundance of HERV-H in microvesicles from GBM cells is consistent with it being the most active HERV in fetal brain cells with these tumours thought to derive from dedifferentiated glia cells or neuroprecursor cells [50] , [51] . The finding of high HERV-K RNAs in several tumour lines is intriguing as this is the most intact of the HERVs in the human genome [52] . Other studies have noted an association between increased retrotransposon activity and tumourigenesis. In some cases, retrotransposon insertion into the genome acts as a driver mutation in tumourigenesis [53] . For example, L1 insertions in oncogenes have occurred in the APC gene in colon cancer [54] and the MYC gene in breast cancer [55] . A potential role for increased retrotransposon activity in tumourigenesis is also suggested by the reduced growth of cancer cells when RT activity is inhibited [56] or when translation of HERV RNAs is blocked by RNA interference [57] . An important question is whether retrotransposon-derived RNA and proteins in tumour microvesicles can be delivered to other cells and contribute to genomic instability. This transfer is supported by our finding of elevated HERV RNA in endothelial cells exposed to tumour microvesicles. Although new retrotransposon insertion events can prove deleterious to cells in some cases [58] , other events could generate cells with increased proliferative or invasive potential. For example, in murine tumours, ongoing endogenous murine leukaemia virus integrations lead to genetic changes implicated in increased cell mobility [59] . Serum microvesicles derived from tumour cells can provide a window into the genotype and phenotype of tumours in individual cancer patients. The exoRNA in serum microvesicles from GBM patients can be used to detect the EGFRvIII mutant/variant mRNA in tumours [8] and elevated miRNAs in ovarian tumours [11] . Further, in the present study, we found that xenograft tumours of human medulloblastoma cells amplified for c-Myc released microvesicles into the serum with elevated expression of c-Myc . Our present findings indicate additional tumour-specific genetic properties represented in microvesicles from tumour cells. First, the exoDNA and exoRNA content is increased in tumour microvesicles as compared with microvesicles from normal fibroblasts, especially, in the case of tumour cells with an amplified oncogene. As DNA is intrinsically more stable than RNA, this should make quantification and analysis of genomic mutations more robust and sensitive in clinical biomarker assays. Elevation of exoDNA or exoRNA may serve as biomarkers of oncogene amplification, for example, c-Myc in individuals harbouring medulloblastoma tumours. Second, increased expression of certain retrotransposon RNAs appears to be a unique feature of tumour cells as compared with normal adult cells. As these retrotransposon sequences are abundant in tumour microvesicles that can be harvested from body fluids, they could be useful as biomarkers. The levels of specific retrotransposon sequences, such as those for specific HERV family members, may be indicative of the cell origin of the tumour [50] . This work expands the list of genetic elements in tumour microvesicles that can potentially be used in blood-based diagnostics for cancer and suggests new modalities of intercellular genetic communication. Cells Primary GBM cell lines 20/3 and 11/5 were generated in our laboratory from tumour specimens kindly provided by Dr Bob Carter (Massachusetts General Hospital), and diagnosed as GBMs by a neuropathologist at Massachusetts General Hospital [8] . GBM cells were cultured in Dulbecco's modified essential medium (DMEM; Invitrogen) containing 10% fetal bovine serum (FBS; JRH Biosciences) and Penicillin/Streptomycin (10 IU ml −1 and 10 μg ml −1 , respectively; Cellgro). Primary medulloblastoma cell lines D458, D384 and D425 were cultured in suspension in DMEM containing 10% FBS, 1×GlutaMAX (Invitrogen) and penicillin/streptomycin. Rhabdoid tumour cell line NS224 (AT/RT) was cultured in DMEM/F12 containing B27 supplement, 20 ng ml −1 epidermal growth factor, 20 ng ml −1 fibroblast growth factor and penicillin/streptomycin. Melanoma cell line, Yumel 0106, was kindly provided by Dr R Halaban (Yale New Haven Hospital, New Haven, CT, USA) and cultured in OptiMEM (Invitrogen) containing 10% FBS and penicillin/streptomycin. Epidermoid carcinoma cell line, A431 (ATCC) was kindly provided by Huilin Shao (Massachusetts General Hospital) and cultured in DMEM containing 10% FBS and penicillin/streptomycin. Human fibroblast lines, HF19 and HF27, were derived from human skin biopsies in the Breakefield laboratory; L2131 was derived in Dr Christine Klein's laboratory (University of Lübeck, Lübeck, Germany) and cultured in DMEM supplemented with 10% FBS, 10 mM HEPES (Invitrogen) and penicillin/streptomycin. HUVECs, kindly provided by Dr Jonathan Song (Massachusetts General Hospital), were cultured in Gelatin-coated flasks in endothelial basal medium (Lonza) supplemented with human epidermal growth factor (hEGF), hydrocortisone, GA-1000 and FBS (Singlequots from Lonza). All cell lines were used over a few passages, as microvesicle yield tended to change over extended passages. Microvesicle isolation Cells were grown in media with 5% microvesicle-depleted fetal bovine serum (dFBS) [8] . Conditioned medium was collected after 48 h and microvesicles were purified by differential centrifugation and filtration through a 0.22 μm filter followed by ultracentrifugation at 110,000× g (ref. 8 ). Microvesicle RNA/DNA extraction Microvesicle pellets generated from 39 ml conditioned medium produced from 0.5×10 6 –3.5×10 6 cells over 48 h were resuspended in 50 μl PBS and incubated at 37 °C for 30 min with DNAse I (DNA-free kit, Ambion) and Exonuclease III (Fermentas), according to manufacturer's recommendation. After treatment, the enzymes were inactivated (using the kit's inactivation reagent and heat inactivation) and samples processed for DNA or RNA isolation. Microvesicles were lysed in 300 μl MirVana lysis buffer (Ambion) followed by extraction with an equal amount of acid-phenol:chloroform. After centrifugation at 10,000× g for 5 min, the upper aqueous phase was removed and further processed to extract DNA and RNA using the Qiagen PCR purification kit or the MirVana RNA isolation kit (Ambion), respectively, according to manufacturer's recommendation. DNA and RNA extracts were then treated with RNAse (RNAse A, Fermentas) or DNAse (DNA-free kit, Ambion) to exclude reciprocal carryover. Quantity and size ranges of exoRNA and exoDNA were evaluated with the 2100 Bioanalyzer (Agilent) using either a RNA 6000 Pico Chip or the DNA 7500 LabChip kit, respectively. S1 nuclease (200 U ml −1 ; Fermentas) was also used to digest single-stranded nucleic acid at 37 °C for 30 min. Nuclear genomic cell DNA was isolated from cells with the Flexigene DNA kit (Qiagen), according to manufacturers' recommendation. qRT-PCR and qPCR Total RNA (50 ng) was converted into cDNA with Sensiscript RT Kit (Qiagen) using random primers, according to manufacturer's recommendations, and a 1:20 fraction (corresponding to 2.5 ng reverse transcribed RNA) was used for qPCR. The gDNA and exoDNA qPCR was carried out using 10 ng DNA as a template. All reactions were performed in a 25 μl reaction using Power SYBR Green PCR Master Mix (Applied Biosystems) and 160 nM of each primer. Amplification conditions consisted of: 1 cycle of 50 °C, 2 min; 1 cycle of 95 °C, 10 min; 40 cycles of 95 °C, 15 s; and 60 °C, 1 min followed by a dissociation curve analysis of each amplicon on the 7000 ABI Prism PCR system (Applied Biosystems). Ct values were analysed in auto mode and manually inspected for accuracy. The Ct values at both RNA and DNA levels were normalized to the housekeeping gene GAPDH in each sample. Primer dimers were excluded by evaluation of dissociation curve and agarose gel electrophoresis. Nanoparticle tracking analysis Microvesicles were purified from all cell lines (D384, D425 and D458, Yumel 0106, GBM11/5, HF19 and HF27). The media was first spun at 300× g for 10 min. The supernatant was removed and spun again at 16,500× g , filtered through a 0.22 μm filter and used for analysis. The Nanosight LM10 nanoparticle characterization system (NanoSight) equipped with a blue laser (405 nm) illumination was used for real-time characterization of the vesicles. The result is presented as the average±s.e.m. of three independent experiments. Xenograft tumour models Two groups of five adult immunodeficient mice (nu/nu NCI) were each injected subcutaneously in both flanks with 5×10 6 medulloblastoma cells (line D425) or epidermoid carcinoma cells (line A431). Tumours were allowed to grow for three weeks; the mice were then killed and blood was drawn by cardiac puncture. Subcutaneous tumour mass weights at the time of euthanization were as follows: D425: 1–3.4 g; 2–1.7 g; 3–2.4 g; 4–2.9 g; 5–1.7 g and A431: 1–1.7 g; 2–2.3 g; 3–3.1 g; 4–1.9 g 5–2.2 g. Approximately 1 ml of blood was obtained from each mouse and allowed to clot at room temperature for 15 min and then centrifuged at 1,300× g for 10 min. The sera was then filtered through a 0.22 μm filter and stored at −80 °C. Samples were thawed and centrifuged for 1 h at 100,000× g to obtain microvesicles for RNA extraction, as described above. All animal procedures were performed according to guidelines issued by the Committee of Animal Care of Massachusetts General Hospital. Estimation of gene copy number by SNP array analysis Genomic DNA was extracted from medulloblastoma cell pellets using the Puregene DNA Extraction Kit (Gentra Systems), according to the manufacturer's instruction. To obtain signal intensities and genotype calls, gDNA samples were digested, labelled and hybridized to Affymetrix 250K StyI SNP arrays, according to the manufacturer's protocol (Affymetrix). Signal intensities were normalized using rank invariant set normalization, and copy numbers for altered genomic regions were inferred using the GLAD (Gain and Loss of DNA) algorithm available in the Genepattern software package ( htpp://www.genepattern.org ). c-Myc copy numbers were inferred by analysing the smoothed copy number data at genomic region ch8q24.12. Microarray comparison of transposable elements in microvesicles versus cells RNA was extracted from microvesicles, as described above. The microarray experiments were performed by Miltenyi Biotec using the Agilent whole human genome microarray (Agilent), 4×44K (44,000 probes), two-color array following the manufacturer's protocol. The array was performed on two different RNA preparations from primary GBM cells and their microvesicles. The microarray data has been deposited in NCBI's Gene Expression Omnibus (GSE13470; GEO, http://www.ncbi.nlm.nih.gov/geo ). MA plots The MA plots for the array data was generated as previously described [42] . The log ratio of the intensities of microvesicle/cell is plotted on the y axis ( M =log 2 Exo–log 2 Cell) and the mean log expression of the two on the x axis ( A =0.5×(log 2 Exo+log 2 Cell)). RT activity assay Microvesicles were lysed in RIPA buffer (50 mM Tris-HCl (pH 8); 150 mM NaCl, 2.5% sodium dodecyl sulphate, 2.5% deoxycholic acid, 2.5% Nonidet P-40) for 20 min at 4 °C. Microvesicle debris was removed by centrifugation at 14,000× g for 15 min. Proteins were quantified by Bradford assay and diluted 1:6 for each RT reaction. The RT assay was performed using the EnzCheck RT assay kit (Invitrogen) on a 25 μl reaction, as described by the manufacturer. Fluorescence signal of the samples was measured before and after the RT incubation. The difference between the two values indicates newly synthesized DNA. Serial dilutions of SuperScript III reverse transcriptase (Invitrogen) were used to generate an RT unit standard curve. The results are presented as the average±s.e.m. of three independent experiments. Microvesicle transfer of HERV-K HUVECs were seeded in 12-well plates at a density of 1.5×10 5 cells per well. Microvesicles were isolated from 1.2×10 7 D384 cells, cultured in dFBS–DMEM, over a 48 h period and added to each well in a total volume of 400 μl DMEM. Mock-treated cells were incubated in 400 μl exosome-free DMEM. The cells were incubated for 2 h at 37 °C and were then replenished with 1.5 ml DMEM (with 5% dFBS). Cells were collected at different time points after the microvesicle exposure and cell RNA was extracted for qRT-PCR analysis. The results are presented as the average±s.e.m. of three independent experiments. Statistics Statistical analyses were performed using the Student's t -test (two tailed). Accession codes: The microarray data has been deposited in the Gene Expression omnibus under accession code GSE13470 . How to cite this article: Balaj, L. et al . Tumour microvesicles contain retrotransposon elements and amplified oncogene sequences. Nat. Commun. 2:180 doi: 10.1038/ncomms1180 (2011).